European sea bass genome and its variation provide insights into adaptation to euryhalinity and speciation The European sea bass ( Dicentrarchus labrax ) is a temperate-zone euryhaline teleost of prime importance for aquaculture and fisheries. This species is subdivided into two naturally hybridizing lineages, one inhabiting the north-eastern Atlantic Ocean and the other the Mediterranean and Black seas. Here we provide a high-quality chromosome-scale assembly of its genome that shows a high degree of synteny with the more highly derived teleosts. We find expansions of gene families specifically associated with ion and water regulation, highlighting adaptation to variation in salinity. We further generate a genome-wide variation map through RAD-sequencing of Atlantic and Mediterranean populations. We show that variation in local recombination rates strongly influences the genomic landscape of diversity within and differentiation between lineages. Comparing predictions of alternative demographic models to the joint allele-frequency spectrum indicates that genomic islands of differentiation between sea bass lineages were generated by varying rates of introgression across the genome following a period of geographical isolation. The European sea bass ( Dicentrarchus labrax ) is a teleost fish found in the north-eastern Atlantic Ocean and throughout the Mediterranean and Black seas. This is an economically important species, and natural stocks are subject to intensive exploitation by professional and sport fisheries, thus raising future conservation and management issues. It is ranked fourth in European aquaculture production and, although undergoing domestication for the last three decades, selective breeding programmes are still in their infancy. The European sea bass inhabits coastal waters, where reproduction occurs; however, it can also enter brackish waters in estuarine areas and coastal lagoons, and occasionally rivers. Thus, the European sea bass is an euryhaline fish tolerating a wide range of salinities (0–60 psu) [1] . Although several genes involved in the physiological response to variation in salinity have been identified [2] , the genetic basis of its broad halotolerance remains unclear. Because adaptation to varying environments may also involve gene duplications [3] , obtaining the complete genome sequence of the European sea bass may help to identify the genetic basis for adaptation to euryhalinity. Atlantic and Mediterranean sea bass populations represent two genetically distinct lineages that naturally hybridize in the Alboran Sea [4] . Describing genomic variation patterns that arise from the interaction between these two diverging lineages has important implications for understanding the evolutionary forces at play during the diversification of marine species. In addition, a detailed picture of genomic variation within and between lineages will provide useful information to orientate domestication and assist conservation management of sea bass populations [5] . Here we produce a high-quality draft sequence of the European sea bass genome by combining high-throughput sequencing with genetic and physical maps [6] , [7] , [8] . The current assembly spans 675 Mbp and contains ~86% of the contigs ordered and orientated along 24 chromosomes, representing one of the highest-quality fish genomes available. Most sea bass chromosomes are highly collinear with those of upper teleosts, confirming the evolutionary stability of fish genomes [9] . We annotate 26,719 genes and identify gene family expansions, some of which are promising candidates for euryhaline adaptation. In addition, we characterize genome-wide variation patterns by restriction-site-associated DNA (RAD)-sequencing ~2.5% of the genome in 100 individuals from the Mediterranean and Atlantic lineages, using three individuals of the congeneric D. punctatus as an outgroup. We find that genomic variation within and between sea bass lineages is influenced by large-scale variation in local recombination rates and by diversifying selection translating into variable rates of introgression across the genome following post-glacial secondary contact. These results provide new insights into the genetic correlates of speciation, as it occurs in a typical marine species with high levels of gene flow and a large effective population size. 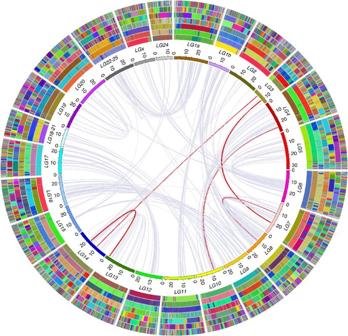Figure 1: Collinear blocks showing the overall degree of synteny between the European sea bass (D. labrax) genome and seven other publicly available teleost genomes represented outside the sea bass chromosomal ring. From the inner to the outer layer:G. aculeatus, O. latipes,T. nigroviridis, D. rerio, O. niloticus,T. rubripesandG. morhua. Sea bass chromosomes (LGn) show conserved synteny with the assemblies ofG. aculeatus, O. latipes,T. nigroviridisandD. rerio, whileO. niloticus,T. rubripesandG. morhuaare still scattered into many ungrouped scaffolds as reflected by tracks of different colours along the chromosomes. The colour code is species-specific. Blocks of collinearity between sea bass chromosomes are represented by grey inner links. Red inner links represent blocks of collinearity containing claudin genes. Genome sequencing and assembly We sequenced the whole genome of a single meiogynogenetic male of the European sea bass to an average coverage depth of 30 × using a combination of whole-genome shotgun, mate pair and BAC end sequencing ( Supplementary Table 1 ). 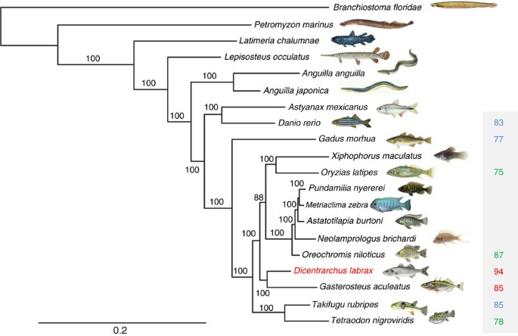Figure 2: Phylogenetic tree based on 621 1:1 high-quality orthologous protein-coding genes from 20 sequenced fish genomes, showing the relationships between European sea bass (D. labrax) and other fish species (half of which belong to the Series Percomorpha). Node support is indicated by bootstrap values. The lancelet (Branchiostoma floridae) was used as the outgroup. The shaded box indicates the total number of gene copies across the five expanded gene families involved in euryhalinity for highly euryhaline (red), euryhaline (green) and stenohaline (blue) species. The reads from three independent sequencing technologies (23.3 Gb) were assembled into a 675-Mb draft genome, with an N50 contig length of 53 kb and an N50 scaffold length of 5.1 Mb ( Supplementary Table 2 ). Using a reference radiation hybrid map [6] , linkage maps [10] , [11] and collinearity with the genome of Gasterosteus aculeatus [12] , we assigned 86% of contig sequences (575 Mb) to 24 chromosomal groups [6] ( Supplementary Table 2 ). Comparison between a previous assembly of three chromosomes [8] and the current assembly resulting from whole-genome sequencing (WGS) revealed high similarities with locally improved scaffold orientation ( Supplementary Fig. 1 ). Genome annotation A combination of ab initio gene prediction, homology search and transcript mapping resulted in 26,719 annotated genes ( Supplementary Tables 3 and 4 ). The 18,253 bp of the whole mitogenome was assembled and annotated, and ranked among the largest in teleost fish ( Supplementary Table 5 ). Repetitive DNA sequences within the sea bass genome accounted for 21.47% of the assembly, with 3.87% of class I transposable elements and 4.19% of DNA transposons ( Supplementary Table 6 ), in line with what has been found in other fish genomes [9] , [13] . 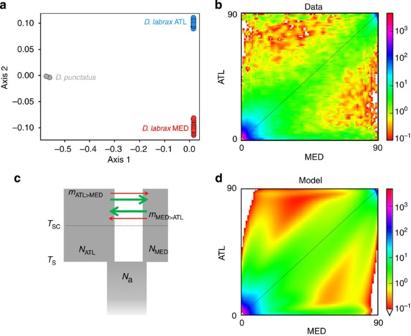Figure 5: Population structure and demographic history of the European sea bass,D. labrax. (a) Principal component analysis of the Atlantic (ATL) and Mediterranean (MED) sea bass lineages including the outgroup speciesD. punctatus.(b) The joint allele-frequency spectrum (AFS) for the ATL and MED populations, showing the count of derived allele for 109,300 oriented SNPs in 45 individuals from each population. (c) The secondary contact with two migration rate model (SC2m), including 10 parameters: the ancestral population size (Na), the ATL and MED population sizes after splitting (NATLandNMED), the splitting time (TS) and the time since secondary contact (TSC). Locus-effective migration rate from ATL into MED (mATL>MED) and in the opposite direction (mMED>ATL) can take two free values in proportionspand 1−p. (d) The maximum-likelihood AFS obtained under theSC2mmodel. Similarly, the average GC content of the sea bass genome (40.4%) was comparable to that of other teleosts [14] . The distribution of GC content was rather homogeneous within chromosomes ( Supplementary Fig. 2 ). We found a lower percentage of GC in noncoding regions (39.6%) compared with protein-coding regions (52.6%), and the third-codon positions GC content was 60.7%, suggesting the effect of selection for codon usage, or a stronger effect of biased gene conversion in coding regions relative to noncoding regions [15] . We found almost complete synteny and large blocks of collinearity between sea bass chromosomes and homologous chromosomes of the three most closely related teleost taxa that have a chromosome-scale assembly ( G. aculeatus, Oreochromis niloticus and Tetraodon nigroviridis ; Fig. 1 and Supplementary Table 7 ). This matches well with the position of sea bass relative to other derived teleosts on a phylogenetic tree reconstructed using 621 1:1 orthologous proteins from 20 sequenced fish genomes ( Fig. 2 ). Our phylogenomic analysis also supports the recently resolved relationships among fully sequenced percomorph fishes, which group sea basses and sticklebacks in a common clade [16] , [17] . Figure 1: Collinear blocks showing the overall degree of synteny between the European sea bass ( D. labrax ) genome and seven other publicly available teleost genomes represented outside the sea bass chromosomal ring. From the inner to the outer layer: G. aculeatus, O. latipes , T. nigroviridis, D. rerio, O. niloticus , T. rubripes and G. morhua . Sea bass chromosomes (LGn) show conserved synteny with the assemblies of G. aculeatus, O. latipes , T. nigroviridis and D. rerio , while O. niloticus , T. rubripes and G. morhua are still scattered into many ungrouped scaffolds as reflected by tracks of different colours along the chromosomes. The colour code is species-specific. Blocks of collinearity between sea bass chromosomes are represented by grey inner links. Red inner links represent blocks of collinearity containing claudin genes. Full size image Figure 2: Phylogenetic tree based on 621 1:1 high-quality orthologous protein-coding genes from 20 sequenced fish genomes, showing the relationships between European sea bass ( D. labrax ) and other fish species (half of which belong to the Series Percomorpha). Node support is indicated by bootstrap values. The lancelet ( Branchiostoma floridae ) was used as the outgroup. The shaded box indicates the total number of gene copies across the five expanded gene families involved in euryhalinity for highly euryhaline (red), euryhaline (green) and stenohaline (blue) species. Full size image Gene duplication and the evolution of euryhalinity We evaluated the evolutionary consequences of gene expansion and differential duplicate gene loss on biological function pathways. Some pathways were enriched within certain chromosomes, including neuroactive ligand-receptor interaction (LG2), cell adhesion molecules (LG13 and LG14), endocytosis (LG19), DNA repair and nucleotide excision repair (LG20). Among the enriched pathways, we detected gene family expansions that may have played a role in adaptation to euryhalinity. These include claudins [18] , [19] , aquaporins [20] , arginine-vasotocin ( AVT ) receptors [21] , prolactin ( PRL ) [22] and its receptor ( PRLR ). Although euryhalinity is an old innovation in aquatic vertebrates that has potentially favoured species diversification [23] , the sea bass genome provides new insights into the genomic modifications at play in this key adaptation. While mammalian genomes have 27 claudins [24] , D. labrax has 61 claudin copies ( Supplementary Fig. 3 ), thus exceeding the 54 copies found in the zebrafish ( Danio rerio ) [25] , which are largely explained by the teleost-specific whole-genome duplication (TGD) [26] . Chromosome blocks containing claudin genes are duplicated in LG13 (15 genes) and LG14 (14 genes) ( Figs 1 and 3 ) and the two claudin clusters of 11 (LG13) and 10 (LG14) tandem genes exhibit conserved synteny to claudins 3 and 4 in human chromosome 7. Expansion of these clusters occurred before the TGD event [26] , since the spotted gar Lepisosteus oculatus has both a single synteny block in LG22 (as in humans) and a tandem cluster of 10 claudins ( Fig. 3 ). However, the coelacanth Latimeria chalumnae has a synteny block with only two claudin genes, indicating an expansion specific to the Actinopterygii lineage occurred [27] . While synteny blocks 1–3 seem to be part of an ancestral chromosome, both Sarcopterygii and Actinopterygii have gained lineage-specific insertions (blocks 4M and 4F) between blocks 1 and 2 ( Fig. 3 ), which appear to have driven claudin expansion both in mammals and teleosts. After the TGD, the teleost-specific duplicate, block 4F on LG14, was translocated between blocks 2 and 3. 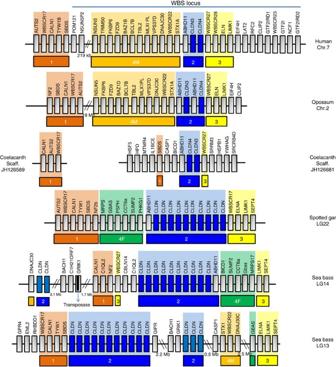The LG13 duplicate, block 4F, was eliminated, while block 3 was translocated to a distant part of the chromosome, blocks 1 and 2 being maintained together. Figure 3: Comparison of claudin gene synteny between sea bass LG 13 and 14 and other vertebrate chromosomes including human. Chromosome blocks containing claudin genes (2) are blue coloured, other synteny blocks are coloured in red (1), yellow (3), orange (4M) and green (4F). Figure 3: Comparison of claudin gene synteny between sea bass LG 13 and 14 and other vertebrate chromosomes including human. Chromosome blocks containing claudin genes (2) are blue coloured, other synteny blocks are coloured in red (1), yellow (3), orange (4M) and green (4F). Full size image The sea bass and zebrafish genomes contain 18 members of the aquaporin family ( Supplementary Fig. 4 ), representing the largest repertoire of functional aquaporins in vertebrates [20] . Both sea bass and zebrafish share duplications of AQP0a-b , AQP1a-b , AQP10a-b and the putative loss of one of the two AQP4 , AQP7 and AQP12 paralogs. However, the AQP5/1 and one of the AQP9 paralogs present in D. rerio are not found in the sea bass. Conversely, sea bass is the only teleost that retains four AQP8 copies as a result of TGD [28] . Teleost genomes contain a large diversity of AVT receptors [21] , with up to six in G. aculeatus , O. niloticus and O. latipes and seven in the sea bass. The latter included duplicated V1A and expansion of V2 from four to five copies, including a novel V2B-like receptor ( Supplementary Fig. 5 ). While the majority of teleosts have maintained single copies of PRL and PRL-like genes, sea bass and Takifugu rubripes [29] retained two PRL-like genes and Oryzias latipes retained two PRL genes ( Supplementary Fig. 6 ). The PRL receptor gene ( PRLR ) is also duplicated in most fish species; however, an extra copy of PRLR-like homolog is present in sea bass, T. rubripes , G. aculeatus and in some cichlids ( Supplementary Fig. 7 ). The sea bass genome has the highest number of gene copies linked to ion and water regulation (94 genes) among fully sequenced teleosts. To test the hypothesis that this gene expansion is associated with the degree of euryhalinity in teleost fishes, a comparison was made to the copy number in the genomes of euryhaline ( T. nigroviridis , O. latipes , O. niloticus and G. aculeatus ) and stenohaline fishes ( D. rerio , Gadus morhua and T. rubripes ); however, no clear pattern was found ( Fig. 2 , Supplementary Table 8 ). However, the analysis of the protein-coding sequences of each gene family showed accelerated evolution of the sea bass PRLR copies one to three and of the novel vasotocin receptor V2B-L , suggesting that relaxed purifying selection or positive selection has occurred for these genes in the lineage leading to sea bass ( Supplementary Tables 9–12 ). Other osmoregulation-related gene duplicates also displayed signatures of positive selection, although not exclusively in sea bass (for example, PRL-L2 ). Altogether, these results suggest that the lineage leading to sea bass has retained a large number of genes involved in ion and volume regulation since TGD, and this may have facilitated the evolution of some genes conferring high tolerance to rapid salinity changes. Searches for recently duplicated genes identified six paralogs that are specific to sea bass, five of which exhibit signatures of positive selection at several amino-acid positions in at least one of the duplicates ( Supplementary Table 13 ). For one of these genes, the nuclear receptor co-activator 5 ( NCOA5 ), sex-differential expression has been reported in Nile tilapia during larval development [30] . Because sex-determining loci in teleosts often involve recently duplicated genes [31] , NCOA5 represents an interesting candidate component of the genetic system for sex determination in sea bass. Genome-wide patterns of polymorphism and recombination A genetic variation map was produced from 100 wild-caught sea bass from the Atlantic Ocean and western Mediterranean Sea. We additionally analysed three spotted sea bass ( D. punctatus ) individuals as outgroup, in order to identify divergent sites between D. labrax and D. punctatus and to polarize single nucleotide polymorphisms (SNPs) within D. labrax ( Supplementary Table 14 ). Genomic variation within and among individuals, lineages and species was examined at ~178,000 RAD tags [32] , providing an average marker density of one pair of RAD tags every 7.5 kb and a 2.5% genome coverage. A total of 234,148 SNPs were found (mean read depth 48 × per individual), revealing an average nucleotide diversity ( π ) of 2.52 × 10 −3 in the Atlantic lineage, 2.60 × 10 −3 in the Mediterranean lineage and 2.31 × 10 −3 in the spotted sea bass. There was broad variation in nucleotide diversity within chromosomes, with a frequently observed fivefold reduced diversity in central chromosomal regions compared with the chromosomal extremities ( Fig. 4a ). Polymorphism was negatively correlated with divergence between D. labrax and the outgroup species D. punctatus ( R 2 =0.085, P <10 −15 ), indicating that the genomic landscape of relative divergence between species was slightly influenced by chromosomal variations in diversity within D. labrax ( Fig. 4b ). Recombination rates were markedly reduced in central chromosomal regions ( Fig. 4c ) and were positively correlated to nucleotide diversity ( R 2 =0.586, P <10 −15 ), while the correlation was negative between recombination and divergence ( R 2 =0.078, P <10 −15 ). Thus, the possible mutagenic role of recombination could not explain the patterns of nucleotide diversity within the sea bass genome, providing evidence for Hill–Robertson effects (including background selection and/or hitchhiking effects) [33] , [34] . Consistent with the effects of selection on SNP variation at a local genomic scale, there was a lower mean expected nucleotide diversity in exonic ( H e =0.067) compared with intronic ( H e =0.075) and intergenic ( H e =0.073) regions. We also observed a diminishing average heterozygosity with decreasing distance to the nearest exon on a very local scale (<200 bp; Supplementary Fig. 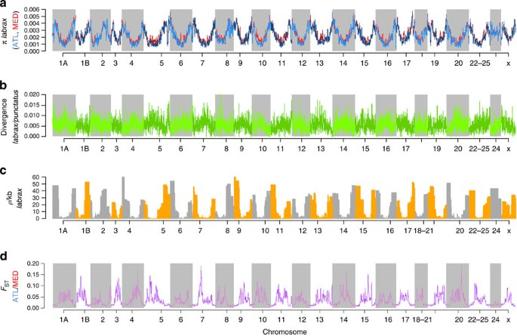8 ), reflecting either Hill–Robertson effects or the direct impact of purifying selection on evolutionarily constrained sites in both coding and cis -regulatory sequences. Figure 4: Distribution of population genetic parameters calculated in 150-kb windows across the different chromosomes of sea bass genome (x refers to LGx, and not to a sexual chromosome). (a) Chromosomal patterns of nucleotide diversity (π) in the Atlantic (blue) and Mediterranean (red) lineages ofD. labrax.(b) Genomic patterns of divergence betweenD. labraxandD. punctatusmeasured as the proportion of fixed differences per bp (df). (c) Chromosomal patterns of recombination (ρ/kb) inD. labrax, averaged across Atlantic and Mediterranean lineages, alternately coloured in grey and orange across chromosomes. (d) Genomic landscape of differentiation (FST) between Atlantic and Mediterranean lineages. Figure 4: Distribution of population genetic parameters calculated in 150-kb windows across the different chromosomes of sea bass genome (x refers to LGx, and not to a sexual chromosome). ( a ) Chromosomal patterns of nucleotide diversity ( π ) in the Atlantic (blue) and Mediterranean (red) lineages of D. labrax. ( b ) Genomic patterns of divergence between D. labrax and D. punctatus measured as the proportion of fixed differences per bp ( d f ). ( c ) Chromosomal patterns of recombination ( ρ /kb) in D. labrax , averaged across Atlantic and Mediterranean lineages, alternately coloured in grey and orange across chromosomes. ( d ) Genomic landscape of differentiation ( F ST ) between Atlantic and Mediterranean lineages. Full size image Genomic landscape of differentiation between lineages Genetic distinctiveness between the Atlantic and Mediterranean lineages of D. labrax was revealed by principal component analysis, in which both lineages appeared equally distant from the closely related spotted sea bass species ( Fig. 5a ). The genome-wide average genetic differentiation between lineages was low ( F ST =0.028) and consistent with previous estimates based on microsatellite markers [4] , [35] , [36] . However, SNP-by-SNP F ST estimates between lineages were heterogeneously distributed across the genome, with highly differentiated markers (some of which reached differential fixation) usually clustering within regions of several hundred Kb to >1 Mb. These genomic islands of differentiation were present in all chromosomes except for LG24 and tended to map disproportionately to central chromosomal regions ( Fig. 4d ). The local averaged F ST was negatively correlated with the local recombination rate ( R 2 =0.257, P <10 −15 ) and nucleotide diversity ( R 2 =0.207, P <10 −15 ), as previously described in other species [37] , [38] . However, a few highly differentiated regions were also found outside low-recombining and poorly polymorphic chromosomal regions (for example, LG13). Therefore, the heterogeneous genomic landscape of differentiation between lineages was only partially explained by the reduced diversity found in the regions of reduced recombination. Figure 5: Population structure and demographic history of the European sea bass, D. labrax . ( a ) Principal component analysis of the Atlantic (ATL) and Mediterranean (MED) sea bass lineages including the outgroup species D. punctatus. ( b ) The joint allele-frequency spectrum (AFS) for the ATL and MED populations, showing the count of derived allele for 109,300 oriented SNPs in 45 individuals from each population. ( c ) The secondary contact with two migration rate model ( SC2m ), including 10 parameters: the ancestral population size ( N a ), the ATL and MED population sizes after splitting ( N ATL and N MED ), the splitting time ( T S ) and the time since secondary contact ( T SC ). Locus-effective migration rate from ATL into MED ( m ATL>MED ) and in the opposite direction ( m MED>ATL ) can take two free values in proportions p and 1− p . ( d ) The maximum-likelihood AFS obtained under the SC2m model. Full size image Demographic divergence history To determine whether and when genomic differentiation patterns were influenced by gene flow, the past demography of European sea bass lineages was inferred using a composite likelihood approach [39] . Seven alternative models of historical divergence were fitted to the joint allele-frequency spectrum of Atlantic and Mediterranean lineages ( Fig. 5b ), including scenarios of strict isolation, isolation-with-migration, ancient migration and secondary contact. The observed allele-frequency spectrum was not satisfactorily reproduced by standard demographic models that assume the gene flow parameter to be shared among loci ( Supplementary Fig. 9 ). A custom secondary contact model with heterogeneous gene flow across the genome [40] ( Fig. 5c ) produced a significantly higher fit compared with all other alternative models ( Fig. 5d ). This analysis revealed several key features of the divergence history of sea bass lineages ( Supplementary Table 15 ). Divergence accumulated during a period of isolation at least 20 times longer than the age of secondary contact. Genetic introgression following secondary contact was strongly asymmetric from the Atlantic to Mediterranean lineage, and occurred at highly variable rates across the genome. We estimated that ~35% of the genome did not freely introgress from one lineage to the other, which mirrors the proportion of the genome in which the windowed F ST lies above the genome-wide average differentiation ( Fig. 4d ). Thus, the genomic islands of differentiation between sea bass lineages appear to have resulted from the erosion of divergence through differential introgression. The European sea bass genome assembly represents one of the first high-quality draft genomes available for an aquaculture fish species and will provide a valuable resource for future evolutionary analyses and genetic improvement. Compared with solely NGS-based genome assemblies, the sea bass genome assembly has benefited from low-coverage Sanger sequencing reads which, combined with data from two different NGS platforms, led to increased contig size. Scaffolding was also improved by combining mate pairs with BAC-end sequences, and a chromosome-scale assembly was obtained using available genetic linkage and radiation hybrid maps anchoring scaffolds to the 24 chromosomes comprising the sea bass karyotype. This genome assembly is a prerequisite to whole-genome or targeted resequencing, RNA-seq, chromatin immunoprecipitation-seq and Methyl-seq experiments, and will therefore catalyse genomic studies in sea bass. In addition, it will help to improve the assembly of newly sequenced genomes from related orders, since large regions of collinearity have been observed with the genome assemblies of other teleost fishes. The sea bass genome sequence may thus facilitate genomic studies in other economically important fishes. Expansions of gene families related to ion and volume regulation were likely mediated through an elevated rate of duplicate gene retention after TGD, providing a genetic basis for adaptation to euryhalinity in the European sea bass and possibly other highly adaptable species. This finding questions the relative importance of whole-genome duplication events versus single-gene duplication in the evolution of euryhalinity in fish, which should motivate broader-scale comparative genomic and experimental studies in the future. The European sea bass also provides an interesting model for understanding the evolutionary mechanisms involved in speciation. Our results imply genetically based reproductive barriers reducing gene flow between Atlantic and Mediterranean sea bass lineages. We reveal important aspects of the genetic architecture of differentiation between these two lineages, such as the disproportionate mapping of the genomic islands of differentiation within low-recombining regions. Evidence for differential gene flow after secondary contact implies that the genomic islands in sea bass are not simply an incidental consequence of reduced diversity in low-recombining regions [41] , but also the product of reduced gene flow in these regions. Furthermore, some genomic islands of high differentiation are also observed in regions of high diversity. Therefore, the genomic landscape of differentiation in sea bass likely results from the preferential erosion of divergence in the genomic regions with high recombination rates. The question of the timing of gene flow has been partly answered by our modelling approach, which dated the secondary contact to ca. 11,500 years BP, and estimated the divergence time to ca. 270,000 years BP (using a per-generation mutation rate of 10 −8 per bp and a generation time of 5 years). This puts the onset of secondary gene flow to the last glacial retreat and strongly supports the role of distributional range shifts caused by Pleistocene glacial periods in promoting divergence. The true evolutionary history is admittedly more complex, since quaternary glacial oscillations may have resulted in intermittent gene flow during divergence. This may explain the contrast between the divergence captured by our analysis of the nuclear genome and the 2.8% divergence found in the nonrecombining mitochondrial genome, which may be involved in old cytonuclear incompatibilities that have remained protected from fixation for a much longer period than the recent history revealed by the coalescence of the rest of the genome. This new picture of the dual origin of the genetic variability in European sea bass brings important data to explain the long-standing observation of genetic discontinuities at the Almeria–Oran front in many marine species [42] . It reinforces the hypothesis of anciently diverged genetic backgrounds being trapped by the Atlantic/Mediterranean environmental boundary [43] , and further supports the role of allopatric isolation as the main driver of marine speciation. Sequencing strategy All sequencing libraries were constructed from the genomic DNA of a single Adriatic sea bass individual (meiogynogenetic male 57) [44] , [45] (kindly provided by the late A. Libertini, CNR, Venice, Italy through J. B. Taggart, University of Stirling, Stirling, UK). The BAC library [44] was obtained from the German Resources Center for Genome Research (RZPD, Berlin, Germany). Plasmid libraries were constructed as previously described [7] . Template preparation was performed automatically at the Max Planck Institute for Molecular Genetics (MPIMG, Berlin, Germany). Purification was based on size-selective precipitation in polyethylene-glycol 6000/2-propanol mixtures [46] . Template DNA was sequenced on ABI3730xl capillary sequencers and raw sequencing data were processed using the PHRED basecaller [47] and LUCY [48] for quality clipping and vector clipping. WGS libraries that were submitted to pyrosequencing were constructed according to the manufacturers’ protocols (Roche) and sequenced on a ROCHE 454 FLX Titanium sequencer. Eight mate-pair libraries of ~20-kb insert size were constructed at 454 Life Sciences (Branford, USA) to support genome scaffolding. For each library, half of a picotiter plate was sequenced on the GS FLX Titanium system. A small-insert library (300 bp) for Illumina sequencing was constructed using the NEBNext DNA Sample Prep Reagent Set 1 (NEB, Ipswich, USA). For the two larger insert libraries (500 and 1,000 bp), only five PCR cycles were performed to reduce amplification bias effects. All libraries were sequenced with 100-bp paired-end runs on an Illumina GAIIx instrument. Genome assembly Before assembly, Illumina sequencing reads were end-clipped to keep the largest part of a read (>64 bp) in which no quality value below 11 occurred. Duplicate reads and residual sequencing adapters were removed. All, 454 reads from 20-kb mate-pair libraries were filtered for duplicates and chimeric mates by mapping them to older assembly versions of the D. labrax genome using gsMapper v2.3 (Roche) and confirming collinearity with G. aculeatus and O. latipes . Sanger reads and 454 single-end reads were directly used for assembly using Celera Assembler v6.1 (CA6.1) [49] . Several softwares for WGS assembly were tested, among which SOAPdenovo (for Illumina data), Newbler (Roche) and CA6.1. CA6.1 was the best-performing one, although the first assemblies needed editing because of inconsistencies in the long-range mate-pair data. These issues were solved by removing duplicates and screening for potential chimeric mate pairs by making use of the strong collinearity of sea bass with the stickleback [12] . After WGS assembly, long-range continuity was improved by re-scaffolding the CA6.1 scaffolds using the BAMBUS scaffolder [50] , including the 454 20-kb mate pairs and BAC ends. These scaffolds were mapped against the G. aculeatus and O. latipes genomes by Megablast. Scaffolds were grouped into sets that were assigned to distinct chromosomal groups in these species to reduce the complexity of chromosome assembly. Finally, markers from the radiation hybrid map [6] , genetic linkage maps [10] , [11] , BAC-end and 454 20-kb mate pairs were mapped on these scaffold groups and CONSED [51] was applied to manually build chromosomal sized superscaffolds. Chromosome names conformed with the naming adopted in the radiation hybrid map. Sequences that could not be ordered into chromosomal groups were concatenated into a superscaffold of unordered genomic pieces (UN). UCSC genome browser of the sea bass genome is at http://seabass.mpipz.mpg.de . Transcriptome sequencing and assembly Paired-end RNA-sequencing was performed using sea bass offspring obtained by crossing wild parents at the Ifremer Station Expérimentale d’Aquaculture (Palavas-les-Flots, France). Four pools of three to four individual liver and intestine total RNA extracts were assembled to prepare four RNAseq libraries of distinct Mediterranean and Atlantic origin ( Supplementary Table 4 ) at the CERBM (Université de Strasbourg, France). mRNA was purified from total RNA using poly-T oligo-attached magnetic beads and fragmented using divalent cations at 95°C during 5 min. After reverse transcription with random primers and ligation to adapters, enrichment was performed through 13 cycles of PCR amplification. PCR products were then purified with AMPure beads (Agencourt). Size selection of ~250–350 bp fragments was performed by electrophoresis on a 2% agarose gel. Libraries were sequenced on four lanes of an Illumina GAIIx using 2 × 100 pb paired-end reads. After library cleaning with Trimmomatic [52] , reads from each of the four lanes were mapped independently on the draft sequence of the sea bass genome with Tophat and then assembled with Cufflinks [53] , and a reference transcriptome was built by merging results of the four lanes with Cuffmerge. Genome annotation The ab initio gene prediction was carried out with GENESCAN [54] . For homology-based predictions, we first mapped known teleost proteins from Ensembl and GenBank databases on the sea bass genome using SPALN aligner v2.12 (ref. 55 ). Custom scripts were used to choose the best-scoring protein match in a cluster of matches defined by exact exon–exon matches in a first iteration and overlapping exons in a second iteration. Second, the CDS models from SPALN were combined with assembled RNAseq data by splitting the gtf files of all predictions and transcripts into overlapping exon–intron–exon fragments and merging them using Cuffmerge [53] . This resulted in a high number of possible transcript models. We used Transdecoder ( http://transdecoder.sourceforge.net ) to assign coding sequences to these models and used the length of the CDS as a score for each model. We weighted the scores of these different models based on their origin (highest rank: RNAseq only, lowest rank: SPALN only). Afterwards, the best-scoring transcript from a cluster of redundant CDS was selected as the reference gene model. Reference genes resulting from our combined annotation were functionally annotated using Blast2GO v2.6.4 (ref. 56 ) and a custom-blast database consisting of vertebrate proteins from GenBank. In additional, the gene model proteins were submitted to InterProScan to identify shared signatures with proteins of known function. Functional annotation of RNAseq data was performed using blastx against Ensembl fish species proteomes and the NCBI nr database. Results were contrasted with annotation based on the direct homology-based method, and permitted annotation of new genes and correction of some gene predictions. Whole-genome alignments Reference genome sequences of seven teleost fishes ( G. aculeatus, O. niloticus, T. nigroviridis, T. rubripes, O. latipes, G. morhua and D. rerio ) were downloaded from the Ensembl website. The LAST tool was applied to produce fast and sensitive whole-genome alignments. We screened for best one-to-one alignments using custom scripts removing repetitive and suboptimal alignments. Blocks of shared collinearity were constructed using the BlockDisplaySatsuma script from the Satsuma v1.17 package [57] . Blocks of collinearity were further combined allowing unaligned regions of up to 100 kb and visualized in the sea bass genome browser. Phylogenetic reconstruction Twenty publicly available genomes were downloaded and formatted as SPALN v2.12 databases. The Ensembl proteins from O. niloticus were used to predict genes in all species by homology using SPALN v2.12. Predicted proteins for each species were filtered to retain only the best-scoring hit to O. niloticus , showing nearly complete coverage and a minimum alignment of 60% of amino-acid residues to an O. niloticus protein. We only retained 621 1:1 orthologous proteins that were found in all 20 genomes. Multiple alignments computed for each protein using ClustalW2.1 were then concatenated and Prottest used to determine the best amino-acid substitution model (JTT I+G) and phyML used to build phylogenetic trees. Other phylogenetic reconstruction methods were also tested (Neighbor Joining, FastTreeMP, MrBayes) and in all trees the nodes were highly supported and only a single difference in tree topology appeared between NJ and the other methods. Visualization of the trees was carried out in TreeDyn. Enrichment pathway analysis Chromosome gene sets were tested for pathway enrichments in comparison with the whole-genome gene set. Sea bass genes were queried against KEGG orthology (KO) database using KOBAS [58] . KO terms of the annotated genes within each sea bass chromosome were used to identify statistically enriched related pathways in chromosomal regions after applying the FDR correction. Detection of gene synteny and collinearity MCScanX’s algorithm was used to perform synteny and collinearity detection across the genome of different species, as well as within the sea bass genome to search for collinear blocks indicative of duplication events and gene family expansions. We used the fraction of collinear genes as a metric to identify collinear blocks. Circular genome representations were created using Circos [59] . Detection of duplicated genes Sea bass-specific gene duplications were detected using a pipeline that interrogates the Ensembl database of orthology groups Compara, using genes from eight teleost genomes to build Compara gene trees ( D. rerio, G. morhua, O. niloticus, T. rubripes, T. nigroviridis, X. maculatus, G. aculeatus and O. latipes ). Putative duplicated genes were then analysed in a rigorous phylogenetic context to assess true orthology. Alignment of protein sequences of all putative orthologues and closely related paralogues in all vertebrates was carried out for each group of duplicates. Amino-acid sequences were aligned using MAFFT [60] under E-INS-I or L-INS-I options. Sequences with insufficient information were discarded. Aligned coding sequences were used to reconstruct a gene tree with PHYML 3.0 (ref. 61 ) using default options. The tree topology was analysed for compatibility with gene duplication occurring in the sea bass lineage. For confirmed duplicated genes, the amino-acid alignment was then transferred into Translator X [62] to guide nucleotide sequence alignment and obtain aligned codon sequences. The tree topology was used as user tree option in the analysis of branch- and site-specific codon evolution, which was implemented in the Data Monkey web server ( http://www.datamonkey.org/ ). Branch Site REL [63] , a branch-specific test for positive selection was used to assess the presence of significantly divergent branches in the gene tree. A mixed effects model of evolution [64] test was used to assess the presence of codons/positions under positive selection. RAD sequencing, SNP discovery and genotyping Wild sea bass individuals were sampled from both the Atlantic Ocean ( n =50) and the western Mediterranean Sea ( n =50), where two distinct lineages have been documented for D. labrax [4] ( Supplementary Table 9 ). Three individuals from the closely related spotted sea bass D. punctatus were sampled in a Tunisian lagoon and used as an outgroup. Genomic DNA was isolated using the DNeasy Blood and Tissue Kit (Qiagen) and digested with Bam HI. Seven RAD libraries were constructed by multiplexing 15 uniquely barcoded individuals per library, following an adaptation of the original protocol [32] . Each library was subsequently sequenced on a separate lane of an Illumina HiSeq2000 instrument with 101-bp single-end reads. Illumina reads were demultiplexed and quality-filtered using Stacks v1.07 (ref. 65 ). Cleaned individual reads were mapped to the reference genome using Bowtie v 2.0 with the very-sensitive option [66] , allowing at most three mismatches per alignment. We then called SNPs from the aligned reads using the Stacks v1.07 pipeline, with a minimum read depth of 5 × per individual per allele to infer individual genotypes. Only RAD loci that were present in at least 70% of the samples in each population were considered for nucleotide diversity analysis. Population genetic analyses Genomic patterns of nucleotide diversity and genetic differentiation were computed in Stacks v1.07 as the weighted average of π and F ST in 150-kb windows [65] . We used a custom script to calculate the mean proportion of fixed differences per bp ( d f ) between D. labrax and D. punctatus in 150-kb windows. SNPs were annotated to exonic, intronic or intergenic regions using SNPdat [67] , and the mean expected heterozygosity in different regions was calculated with VCFtools v0.1.11 (ref. 68 ). Variable recombination rates along each chromosome ( ρ =4 N e r per kb) were estimated using a Bayesian reversible-jump MCMC scheme under the crossing-over model of interval in LDhat [69] , with 10 million iterations and 5 million burn-ins. Population structure was examined using a principal component analysis in SNPRelate [70] . The demographic history of Atlantic and Mediterranean sea bass populations was inferred from their joint site frequency spectrum (SFS) in δaδi v1.6.3 (ref. 39 ). We used 109,329 SNPs that were polymorphic in D. labrax but fixed in D. punctatus to determine the most parsimonious ancestral allele in D. labrax . The joint SFS was projected to 45 individuals in each population to avoid missing genotypes. We considered seven alternative models of historical divergence: Strict Isolation ( SI ), Isolation-with-Migration ( IM ), Ancient Migration ( AM ), Secondary Contact ( SC ) and their heterogeneous migration rates versions: IM2m , AM2m and SC2m ( Supplementary Fig. 9 ). How to cite this article : Tine, M. et al. European sea bass genome and its variation provide insights into adaptation to euryhalinity and speciation. Nat. Commun. 5:5770 doi: 10.1038/ncomms6770 (2014). Accession codes. Sequencing reads have been deposited in the GenBank/EMBL/DDBJ Sequence Read Archive under the accession codes CBXY010000001 to CBXY010037781 (for Contigs) and HG916827 to HG916851 (for chromosomal scale assembly). Mitochondrial genomes for D. labrax Mediterranean, D. labrax Atlantic and D. punctatus have been deposited in GenBank/EMBL/DDBJ under the accession codes KJ168065 , KJ168064 and KJ168066 , respectively.